Protein design with a comprehensive statistical energy function and boosted by experimental selection for foldability The de novo design of amino acid sequences to fold into desired structures is a way to reach a more thorough understanding of how amino acid sequences encode protein structures and to supply methods for protein engineering. Notwithstanding significant breakthroughs, there are noteworthy limitations in current computational protein design. To overcome them needs computational models to complement current ones and experimental tools to provide extensive feedbacks to theory. Here we develop a comprehensive statistical energy function for protein design with a new general strategy and verify that it can complement and rival current well-established models. We establish that an experimental approach can be used to efficiently assess or improve the foldability of designed proteins. We report four de novo proteins for different targets, all experimentally verified to be well-folded, solved solution structures for two being in excellent agreement with respective design targets. In recent years, protein design has achieved some milestone successes with profound implications in biosciences and biotechnology [1] , [2] , [3] , including the designs of a novel protein fold [4] , new biomolecular interactions and regulations [5] , as well as new biocatalysts [6] , [7] . These progresses have been driven by underlying computational or rule-based design methods, which can be stringently calibrated through the de novo design of amino acid sequences that fold into desired three-dimensional structures [4] , [8] , [9] , [10] . In this regard, rule-based designs have attained some remarkable successes [7] , [11] , [12] , albeit limited to particular types of target structures or structure motifs. More general methods such as RosettaDesign [13] are based on minimizing an effective energy function, which has been, for large parts, derived from molecular mechanics force fields [4] . It has been shown that RosettaDesign can achieve high success rates for idealized target structures [10] . However, success rates of automated design with common targets has remained low [14] , [15] . Meanwhile, different sequences designed for the same target are usually highly homogeneous, not reflecting the diversity of natural sequences sharing conserved structures [15] . In many cases, the designed proteins also lacked the rich conformational dynamics exhibited by their native counterparts [16] . Given the great promises held by protein design, it will be of wide impact to improve computational protein design from its current level. This is especially challenging given that substantial method improvements have not been seen for a decade despite intensive research efforts. It may require novel theoretical approaches that can complement current best methods. Method improvements can also be tremendously accelerated by experimental tools that can yield extensive feedbacks to theory by, for example, distinguishing between positive and negative design results rapidly, as well as telling what might be the design errors and suggesting how to correct them [15] . Conventional in vitro structure analysis augmented by site-directed mutagenesis can barely do the job because of its low throughput and high costs. Although efficient experimental methods may be devised for target proteins with specific selectable functions [17] , a generally applicable approach is yet to be established [15] . The first aim of this work was to develop and validate a comprehensive energy function with novel ingredients so that it could verifiably complement current models of computational protein design. We considered statistical energy functions (SEFs), which were derived from known sequence and structure data of natural proteins [18] , [19] . Potentially, an SEF may pick up factors in protein sequence–structure relationships that are not yet treated properly by current physics-based models. Although SEFs for protein structure prediction have been well developed [20] , [21] and most current protein design approaches contain certain statistical terms [4] , [13] , a comprehensive or full-scale SEF that by itself achieves automated protein design has not been established to compete with state of the art physics-based models [22] . In most previous SEFs, probability distributions were estimated based on a prior discretization of structural properties, for example, the solvent accessibility partitioned into a few discrete categories, or a distance divided into bins. Although sensible for SEFs aimed at structure prediction, this approach leads to several problems for sequence design. First, some target properties will fall near not the centre but the boundary of pre-defined intervals, causing significant biases in probability estimations. Second, it is difficult to treat multiple and/or multi-dimensional properties jointly with decent accuracies. Here we propose a general strategy of selecting structure neighbours with adaptive criteria (SSNAC) to address these accuracy-jeopardizing issues. In this approach, conditional distributions of single or pairs of amino acid types are estimated from training data selected as neighbouring items centred on a target point in a space spanned by multiple structural properties, allowing straightforward considerations of different types of structural properties as joint conditions for the distributions. Adaptive cutoffs for training data selection are used to balance between the amount and the relevance of the training data. A special likelihood-range-based procedure was devised to correct the effects of small sample size. How the various structure properties are selected and treated for the single residue and the residue pairwise SEF terms are determined based on redesigning single sites in native proteins. The resulting pure SEF (noted as E SEF ) treats inter-residue side-chain packing at a highly coarse-grained level. Its extension to include van der Waals energies (noted as E SEF_v ) to treat finer packing effects has also been considered. Our second aim was to establish the applicability and efficiency of an experimental method to assess and/or to correct de novo designed proteins. This approach was originally developed by Foit et al. [23] to evolve protein stability in vivo . In the approach, the structural stability of a protein of interest (POI) is linked to the antibiotic resistance of bacteria cells expressing an engineered TEM1-β-lactamase that contains the POI with flanking linker sequences composed of a few tens of glycine/serine residues as an inserted segment. POIs that are not well-folded are prone to proteolysis by periplasmic proteases specifically recognizing unfolded proteins, leading to weak antibiotic resistance of host cells. This system may be used not only to assess the foldability of designed proteins but also to select mutations that can rescue an initially problematic design. Such results may comprise critical feedbacks for the improvement of computational models and are not easily obtained through other approaches. In this work, we construct an SEF based on the SSNAC strategy and compare it with the established method of RosettaDesign [13] in fixed backbone design. Redesigned sequences for 40 native protein backbones covering different fold classes are evaluated by ab initio structure predictions and energy analyses. The TEM1-β-lactamase-based selection is applied to several designed proteins followed by nuclear magnetic resonance (NMR) analysis. Four well-folded de novo proteins for three different targets are obtained, one having exactly the designed sequence and the other three containing a few point mutations. Solution structures of two de novo proteins are solved by NMR and they are in excellent agreement with respective design targets. These results suggest that the SEF may complement and rival established models for computational protein design. Sequences designed with it can be well-folded or close to foldable. In addition, the TEM1-β-lactamase-based system is highly efficient in assessing and improving the foldability of de novo proteins. Theoretical tests of the SEF We first tested the SEFs theoretically. Design targets were 40 backbone structures of 76–191 residues from the Protein Data Bank (PDB), spanning 4 structure classes (all-α, all-β, α/β and α+β) according to the structure classification of proteins [24] . For each target, we designed three sequences using the SEF developed here. For comparisons, another three sequences were designed using Rosetta fixed backbone design. 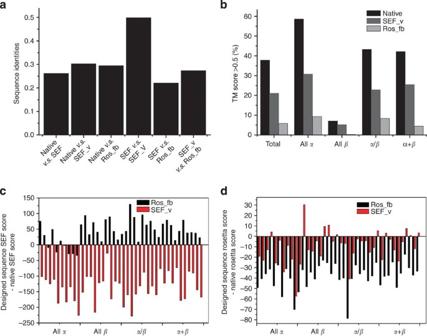Figure 1: Complementarity between SEFs and physics-based energy functions. (a) Sequence identities between native proteins, proteins designed with SEF, proteins designed with SEF_v and proteins obtained with Rosetta fixed backbone design (Ros_fb). Results are averages over 40 target proteins. (b) Fractions of highly target-like models in structures predictedab initiousing native and using different designed sequences. The fold classes of targets are indicated. For each fold class, results are averages over ten targets. (c) Energies of designed sequences relative to corresponding native sequences for 40 target proteins of different fold classes. The energies were calculated withESEF. (d) Same as inc, but the energies were calculated with Rosetta. Target PDB IDs are given in Supplementary Table 1 and the designed sequences in Supplementary Tables 12–14 . Despite the fact that our SEFs do not contain any residue type-specific constant reference energy terms, designed sequences are of overall amino acid compositions similar to native proteins ( Supplementary Table 5 ). The SEF or SEF_v design results have sequence identities of about 30% relative to respective native proteins, similar to sequences produced with Rosetta fixed backbone design ( Fig. 1a ). Figure 1a also shows that the sequences designed with the SEFs have lower than 30% sequence identities with those designed with Rosetta fixed backbone. As would be expected, the sequence identities are lower for surface positions than for those less solvent-exposed positions ( Supplementary Table 6 ). Thus, for the same target structure, the low energy sequences of the current SEF can diverge significantly from those of RosettaDesign, indicating mutual complementary of the two approaches in their solution spaces. Figure 1: Complementarity between SEFs and physics-based energy functions. ( a ) Sequence identities between native proteins, proteins designed with SEF, proteins designed with SEF_v and proteins obtained with Rosetta fixed backbone design (Ros_fb). Results are averages over 40 target proteins. ( b ) Fractions of highly target-like models in structures predicted ab initio using native and using different designed sequences. The fold classes of targets are indicated. For each fold class, results are averages over ten targets. ( c ) Energies of designed sequences relative to corresponding native sequences for 40 target proteins of different fold classes. The energies were calculated with E SEF . ( d ) Same as in c , but the energies were calculated with Rosetta. Full size image We applied Rosetta ab initio structure prediction [25] to each designed sequence and each native sequence. In ab initio structure prediction, tertiary structure models of input sequences are constructed without using any native protein tertiary structures as templates. The similarity of predicted models with corresponding design targets were quantified using the template modeling score or TM score [26] , a quantity to measure structure similarity with a numerical value from 0 to 1. For each sequence, 200 structures were predicted. Statistics of the TM scores for individual targets are reported in Supplementary Table 7 . The results for targets of different fold classes are summarized in Fig. 1b (the results for SEF_v are shown in this figure, the results for SEF being similar, see also Supplementary Table 7 ). According to these data, the sequences designed using our SEF do not, in general, lead to as high fractions of highly target-like predicted models (TM score >0.5) as the native sequences; however, they significantly surpass the Rosetta fixed backbone design results, especially for targets containing β-strands, although the prediction method itself also has worse performance on these targets than on the all-α ones. It seems that the major cause for the Rosetta sequences to lead to worse predicted tertiary structures is not their poorer secondary structure propensities. We carried out secondary structure predictions on the native and the designed sequences, and checked their agreement rates with targets. For the Rosetta sequences, this agreement rate averaged over all 40 targets is still 81%, to be compared with the average rate of 83% for the native sequences and 86% for the SEF sequences. In addition, for quite a number of targets for which the Rosetta-designed sequences do lead to high rates (above 85%) of correctly predicted secondary structures, the predicted tertiary structures still agreed much poorer with respective targets than the same predictions for the native or the SEF sequences. To further examine the complementarity between different energy functions, we separately applied the Rosetta energy function and the SEF to evaluate the energies of sequences deigned with E SEF_v and with Rosetta fixed backbone, respectively, both under corresponding target structures. The energies were compared with those calculated for the native sequences using the same energy functions ( Fig. 1c,d ). As expected, calculated with the Rosetta/SEF energy function, the sequences designed by Rosetta/SEF_v have lower energies. Interestingly, the Rosetta energy function predicts that the sequences designed by SEF_v have lower energies than the corresponding native sequences. Surprisingly, the SEF predicts that most of the results of Rosetta fixed backbone design for the non-all-α targets have significantly higher sequence energies than the corresponding native sequences. Thus, the SEF captures certain energy contributions that favour the native sequences over the Rosetta fixed backbone designs. Assuming that the native sequences are indeed more compatible to respective target structures either according to ab initio structure prediction or based on the fact that the native sequences are known for sure to fold into respective target structures, this result suggests that these energy contributions may be missed or insufficiently represented in current state-of-the-art energy functions for computational protein design. Decomposing the total energy differences into components ( Supplementary Tables 8 and 9 ) suggests that the pairwise SEF terms play important parts. Although a statistical pairwise term in the Rosetta energy function favours the Rosetta-designed sequences over the native sequences for all target classes ( Supplementary Table 8 ), the pairwise term in the current SEF does the opposite, except for the all-α classes ( Supplementary Table 9 ). Enabled by the SSNAC strategy, the present model specifies the structural characteristics of interacting position pairs much more completely than previous statistical models. Experimental assessment and evolution of designed proteins Several proteins designed with E SEF or E SEF_v were experimentally characterized with the TEM1-β-lactamase-based in vivo system as well as with solution NMR spectroscopy. For the examined sequences, antibiotics resistance conferred by corresponding fusion proteins ( Fig. 2a ) well correlate with the propensity of the designed proteins to form well-folded structures in solution as suggested by NMR spectra ( Fig. 2b ): three designed proteins, D_1cy5, D_1r26 and Dv_1r26 lead to weak antibiotics resistance, while the corresponding 1 H-NMR spectra also do not suggest unique well-folded structures; another designed protein, Dv_1cy5, leads to an intermediate level of antibiotics resistance, while its 1 H-NMR spectrum do signal folded structures; the designed protein Dv_1ubq leads to strong antibiotics resistance, in consistence with its 1 H-NMR spectrum strongly signalling a stable structure. 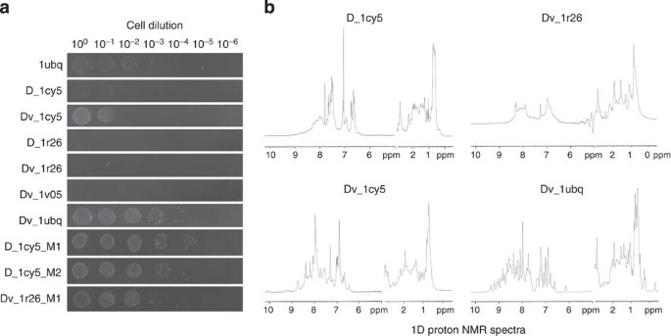Figure 2: TEM1-β-lactamase antibiotic resistance correlates with the foldability ofde novoproteins. The designed proteins are named as ‘D_X’ for those designed withESEF, or ‘Dv_X’ for those designed withESEF_v, the symbol ‘X’ to be replaced by the PDB ID of respective targets. Mutants of designed proteins are named with the extra ‘_Mn’ attached to the names of original proteins, with ‘n’ being a numerical ID. Native ubiquitin is labelled as ‘1ubq’. (a) Antibiotic resistance associated with various proteins. (b)1H-NMR spectra ofde novodesigned proteins. Figure 2: TEM1-β-lactamase antibiotic resistance correlates with the foldability of de novo proteins. The designed proteins are named as ‘D_X’ for those designed with E SEF , or ‘Dv_X’ for those designed with E SEF_v , the symbol ‘X’ to be replaced by the PDB ID of respective targets. Mutants of designed proteins are named with the extra ‘_Mn’ attached to the names of original proteins, with ‘n’ being a numerical ID. Native ubiquitin is labelled as ‘1ubq’. ( a ) Antibiotic resistance associated with various proteins. ( b ) 1 H-NMR spectra of de novo designed proteins. Full size image For two of the initially designed sequences (D_1cy5 and Dv_1r26) that were not associated with strong antibiotic resistance and did not exhibit well-folded structures, we carried out directed evolution of their foldability, again using the TEM1-β-lactamase-based in viv o system. After one or two rounds of selection, several mutants that led to strong antibiotic resistance were identified. Some of them were further characterized by 1 H-NMR spectroscopy (results not shown), based on which three mutants (D_1cy5_M1, D_1cy5_M2 and Dv_1r26_M1, for their associated antibiotic resistance see Fig. 2a ) were selected for subsequent 1 H– 15 N heteronuclear single quantum coherence experiments. The results ( Fig. 3a–c ) proved that these mutants ( Fig. 3d,e ) indeed form well-folded three-dimensional structures. 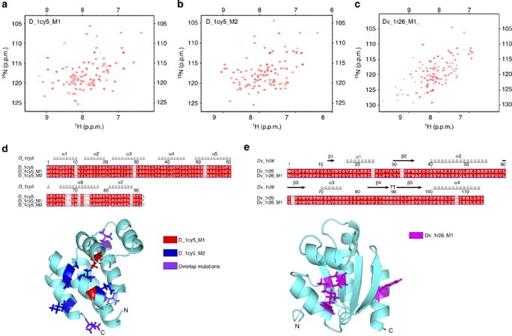Figure 3: Well-folded mutants obtained by directed evolution. (a–c)1H–15N NMR heteronuclear single quantum coherence (HSQC) spectra of different well-folded mutants. (d) Types and locations of mutations in D_1cy5_M1 and D_1cy5_M2. Target secondary and tertiary structures are shown. Sticks represent original side chains at mutated positions. (e) Same as ind, but for Dv_1r26_M1. Figure 3: Well-folded mutants obtained by directed evolution. ( a – c ) 1 H– 15 N NMR heteronuclear single quantum coherence (HSQC) spectra of different well-folded mutants. ( d ) Types and locations of mutations in D_1cy5_M1 and D_1cy5_M2. Target secondary and tertiary structures are shown. Sticks represent original side chains at mutated positions. ( e ) Same as in d , but for Dv_1r26_M1. Full size image Differential scanning calorimetry (DSC) was employed to measure the melting temperatures of these proteins. The melting temperatures (measured as peak positions on respective relative-specific heat versus temperature curves, see Supplementary Fig. 1 ) are 123.3 °C for Dv_1ubq, 84.8 °C for D_1cy5_M1, 58.3 °C for D_1cy5_M2 and 74.0 °C for Dv_1r26_M1. The DSC curve of Dv_1ubq suggests that this protein is highly thermostable. For the other three proteins, respective DSC results suggest that their thermo unfolding is not very cooperative. Temperature-dependent circular dichroism (CD) spectra of the proteins were also measured ( Supplementary Fig. 2 ). The CD spectra are consistent with expected secondary structure types and contents of respective proteins. They are consistent with the DSC results as well. The CD spectrum of Dv_1ubq does not show much change with increased temperature. For the other three proteins, the CD results suggest insignificant and non-cooperative loss of secondary structures at high temperatures. Such thermo-unfolding behaviours are often encountered in designed proteins [27] , [28] , [29] irrespective of energy functions or rules used during design. It could be results of the shared design strategy of stabilizing the folded structures as much as possible in all aspects according to the given energy functions or rules. The data indicate two things: first, some de novo designed proteins, although not exactly being foldable, are in fact very close to foldable ones in the sequence space; and second, the TEM1-β-lactamase-based in vivo system can make a highly efficient method for finding out whether the initially problematic designs can be rectified through sequence perturbations, and how. As such data accumulates, pitfalls in design methods may be revealed for subsequent analysis and improvement. Solution structures of two de novo proteins We carried out necessary NMR spectroscopy experiments to determine the solution structures of Dv_1ubq and D_1cy5_M2. The sequence of Dv_1ubq has been designed with the SEF_v energy function using the structure of human ubiquitin as target (PDB ID 1ubq). The solution structure of Dv_1ubq is highly similar to 1ubq ( Fig. 4a ), the root mean square deviation (RMSD) of α C atom positions between the two structures being 1.17 Å. In Dv_1ubq, 51 of the total 76 amino acid residues have been changed from those in 1ubq (we note that the Dv_1ubq residues identical to those in 1ubq were not pre-fixed but also generated by design). Thus, most of the tertiary inter-residue contacts in 1ubq, although still maintained in Dv_1ubq, have been substituted by contacts between different types of residue pairs ( Fig. 4b ). To examine the overall effects of the completely computer-designed sequence changes on structure stability, guanidine hydrochloride-induced denaturation experiments were performed on both the native and the designed proteins. The results suggested that the designed protein Dv_1ubq is structurally more stable than its native counterpart 1ubq ( Fig. 4c ). 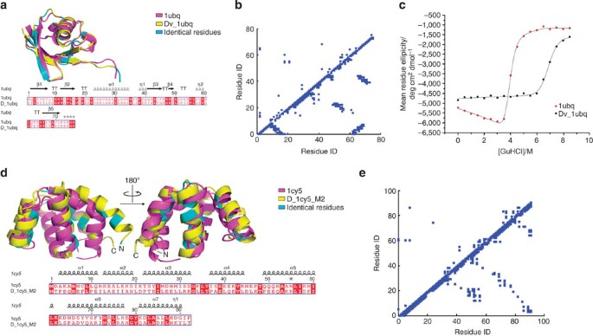Figure 4:De novoproteins compared with native ones. (a) Sequence and structure of Dv_1ubq compared with those of 1ubq. The distribution of identical residues is indicated. (b) Tertiary inter-residue contacts of Dv_1ubq compared with those of 1ubq. The upper triangle of the contact map shows contacts that are the same (that is, formed by the same two types of residues) in the two proteins. The lower triangle shows the remaining contacts. (c) Results of CD in induced denaturing of designed Dv_1ubq compared with native ubiquitin. (d,e) Same as ina,b, but for comparisons between D_1cy5_M2 and 1cy5. Figure 4: De novo proteins compared with native ones. ( a ) Sequence and structure of Dv_1ubq compared with those of 1ubq. The distribution of identical residues is indicated. ( b ) Tertiary inter-residue contacts of Dv_1ubq compared with those of 1ubq. The upper triangle of the contact map shows contacts that are the same (that is, formed by the same two types of residues) in the two proteins. The lower triangle shows the remaining contacts. ( c ) Results of CD in induced denaturing of designed Dv_1ubq compared with native ubiquitin. ( d , e ) Same as in a , b , but for comparisons between D_1cy5_M2 and 1cy5. Full size image The sequence of D_1cy5_M2 has been obtained by completely redesigning the sequence of human caspase recruitment domain (PDB ID 1cy5) with the SEF energy function, followed by antibiotic resistance-based in vivo selection of fold-stabilizing mutations ( Figs 2a and 3b ). The structure of D_1cy5_M2 is in good agreement with that of 1cy5, the target for designing the parent sequence D_1cy5. Both structures have the same six helix–helix bundle fold with the Greek key topology. The major difference between the two structures is limited to a short amino-terminal segment: in 1cy5, the first helix (residues 3–19) is kinked around residue 12, resulting in 2 helix segments (labelled as α 1 and α 2 , respectively, above the 1cy5 sequence shown in Fig. 4d ) forming an angle of about 141°; in D_1cy5_M2, the kink around residue 12 is much less obvious, resulting in an intact helix which is almost straight ( Fig. 4d ). The N-terminal segment (residues 1–11) excluded the remaining parts of the two proteins (residues 11–89) can be well superimposed ( Fig. 4d ) with a α C atom position RMSD of 2.35 Å. We note that Dv_1ubq fold into its desired target structure more closely than D_1cy5_M2. This might have been caused by that Dv_1ubq has been designed with an additional van der Waals energy component that treats atomic packing in a more fine-grained manner than the SEF alone. On the other hand, it might also be due to that the α/β ubiquitin fold adopted by Dv_1ubq and 1ubq is intrinsically less dynamic than the all-α-death-domain fold adopted by 1cy5 and D_1cy5_M2. In D_1cy5_M2, 69 out of its total 92 residues are different from those in 1cy5. Thus, most of the inter-residue tertiary contacts are also formed by different types of residue pairs in these two proteins ( Fig. 4e ). Although the exact designed sequence D_1cy5 is not yet able to fold (which is unlike the case of Dv_1ubq), the agreement between the structures of D_1cy5_M2 and 1cy5 strongly testifies on the accuracy of the SEF to design D_1cy5, the parent sequence of D_1cy5_M2. In summary, we proposed a novel strategy to construct SEFs for protein design and built a comprehensive SEF based on this strategy. Ab initio structure prediction and sequence energy comparisons suggest that the SEF can complement and rival current well-established physics-based models. We found that the TEM1-β-lactamase-based in vivo system was well suited both to directly assess the foldability of designed sequences and to identify foldable sequences close to initial designs. As examples, we have obtained four de novo proteins for three target structures, all experimentally verified to be well folded. We reported solution structures for two of these proteins, one having exactly the designed sequence and the other being a mutant of an initial design, with the mutations identified through efficient directed evolution. Both structures are in excellent agreement with respective design targets. In a certain sense, protein design with SEFs shares spirits with rule-based protein design approaches. However, the descriptive rules one may actually use to design a protein sequence are very few, having been discovered only unsystematically, and definitely being far from complete. To make the situation worse, one usually does not know how to balance between different rules when they are in conflicts with each other. Thus, rule-based designs strongly rely on human expertise and have so far been successful only for special secondary structure motifs or special topologies (for example, helix bundles). In the SEF constructed with the SSNAC strategy, the ‘rules’ have been extracted in a systematic way and integrated in a coherent manner. Compared with previous SEFs or statistical components in an overall energy function, our SEF contains a number of novel ingredients that may be of key importance for its improved accuracy. First, each of the one-residue and two-residue distributions are conditioned on multiple structural properties jointly, not separately. The differences between these two types of treatment are profound. As an example, we assume that the rotamer preference at a position i is dependent on two types of structure properties, one being the secondary structure type and the other being the solvent accessibility. When the two types of property are considered jointly, we have a single one-residue SEF energy term, namely, E i ( r i )=−ln P ( r i |{ SS i , SA i }). On the other hand, when the two types of property are considered separately, the one-residue SEF energy would be the sum of two terms, namely, E i ( r i )=−ln P ( r i | SS i )−ln P ( r i | SA i ). The two different formulations lead to different statistics. If the effects of secondary structure and solvent accessibility on sequence preferences were strongly coupled (and they probably are), the first formulation would be much more accurate. In fact, the large difference between the two treatments can be seen from the single-site redesign results (see Method and Supplementary Method ) comparing different forms of the pairwise SEF terms ( Supplementary Table 3 ). In one form, the relative positioning of two residues were considered independently from local structural properties of individual residues (corresponding results are in the row entry 0_0_0_0.5 of the table). The resulting pairwise SEF terms can barely improve over the SEF with only the single-residue terms but no pairwise terms (compare results in Supplementary Table 3 with those in Supplementary Table 2 ). For comparisons, the remaining results in Supplementary Table 3 indicate that the jointed consideration of relative positioning and local structural properties brought about large improvements. The joint consideration of multiple structural properties in individual SEF terms is straightforward in the construction of SEF terms based on structure neighbours. We note that Keating and coworkers [30] have used pairwise SEF terms based on structure neighbours. A conceptual difference between our work and theirs is that the coupling of inter-residue geometries with one-residue local structural properties has been considered in our work but not in theirs. Another practically important difference is that in ref. 27 the criterion for structure neighbours was based not on RMSD but on inter- α C atom and inter- β C atom distances. We expect the RMSD parameter to specify structure similarity much more thoroughly. In fact, the RMSD-based and the distance-based methods select very different training residue pairs for the same pair of target backbone positions. With the residue pairs in the target 1ubq as examples, training pairs selected using our criteria (RMSD and local structural properties considered jointly) and those selected using the criteria in ref. 30 are only <2% in common. In the meanwhile, the distance-based approach needed a rather restrictive or target-structure-sensitive cutoff (deviations in both distances below 0.1 Å), while the RMSD criterion with the chosen (adaptive) cutoffs is much more inclusive. If the distance-based criterion in ref. 30 were also considered jointly with local structural properties, the number of selected training pairs would be an order of magnitude less than those selected by the RMSD criterion, common training pairs being still only a few per cent. The price for considering multiple structure properties as joint conditions is that the amount of selected training data can be reduced significantly. This may lead to large statistical uncertainties. The situation can be especially severe for the rotamer-based pairwise SEF terms because of the large size of the variable space (that is, there are several thousands of possible rotamer-type combinations over which pairwise distributions need to be estimated). The remaining two novel ingredients in our SEF approach address this problem. One is the adaptive adjustment of selection criteria for training data. In the single-site redesign experiments, this treatment brought about only moderate improvements in the averaged results ( Supplementary Table 3 ). However, if we consider that using adaptive criteria will only affect sites for which insufficient training data could be selected by the more stringent criteria, the moderate improvements reflected by the results averaged over all sites actually indicate substantial improvements for a relatively small number of sites. Another ingredient in our method to diminish the negative impacts of reduced training data is the special scheme of obtaining final probability estimations by weighing observed distributions with respect to background distributions based on likelihood ranges (see Methods). With this empirical scheme, even when the sample size (that is, the number of selected training pairs) is comparable to or even smaller than the size of the variable space (for example, the number of possible rotamer-type combinations), dominating terms of the probability distributions (for example, larger probabilities associated with pairs of rotamer types that are especially favoured) may still be estimated reasonably well. As atomic coordinates have been used in the RMSD-based SEF terms, one question to raise would be how sensitive the resulting SEF is to the quality or accuracy of the backbone coordinates of the target. Several observations suggest that the SEF should be applicable to target backbone coordinates of moderate accuracy, such as those generated not from high-resolution X-ray crystallography but by current computational modelling techniques. One observation is that the (adaptive) RMSD-based criterion is inclusive enough so that every pairwise SEF term can draw information from a large number of interacting residue pairs from diverse protein structures. In Supplementary Fig. 3 , we have shown for the pairwise SEF terms of target 1ubq the distribution of number of training residue pairs and the distribution of number of training proteins contributing the training pairs. The broad training data should cover a wide range of structure variations. Thus, the SEF constructed from them should not be very sensitive to small variations or inaccuracies in target backbone coordinates. Just to obtain some ideas on this issue, we have used modelled homologous backbones of 1ubq as targets to design new sequences (see captions of Supplementary Figs 4 and 5 , the RMSDs between the modelled and the X-ray backbones are around 1 Å). Although the designed sequences did show some degrees of target-induced variations (pairwise sequence identities >80% between sequences designed for the same backbone and 50 ∼ 60% between sequences designed for different target backbones), the sequence logos generated from different sets of designed sequences show highly similar positions and types of conserved residues types throughout the entire sequence ( Supplementary Figs 4 and 5 ). We would like to note that the current SEF should not be confused with methods that use sequence profiles constructed from natural protein templates with overall sequence or structure similarity to design targets [31] . As results, the SEF can be applied to general target structures in different fields of protein engineering, either to design specific sequences or to design highly focused sequence libraries. We note that the current SEF itself does not yet treat atomic packing in the same level of details as physics-based models such as RosettaDeisgn. However, it seems to do a much better job than current physics-based models in capturing the overall topology-related features of protein sequences, especially for β-strand-containing topologies. In addition, the two types of models explore in different regions of the sequence space. Thus, they highly complement each other in a number of important aspects. The fact that either type can now accomplish fully automated design for general targets suggest that integrating them tightly together may substantially boost the accuracy of computational protein design from its current level. In addition, the in vivo experimental approach we used to assess and improve the foldability of designed proteins offers an option of much higher efficiency and far less costs than conventional structure analysis. It may be able to provide extensive feedbacks on both positive and negative design results. Such results are much-needed for continuous method improvement. These progresses may accelerate the development of computational protein design into a robust tool for a wide range of challenging applications. Components of the SEF These includes single-residue terms and pairwise terms, namely, where L is the length of the target peptide chain, i and j indicate positions along the chain. The variable r i with i between 1 to L can denote a residue type or, more generally, it can denote a rotamer type that specifies besides a residue type a discrete side-chain conformational state. The individual terms E i ( r i ) and E ij ( r i , r j ) are determined by the probability distributions of rotamer types and pairs of rotamer types, respectively, conditioned on the structural properties associated with the corresponding position or pair of positions along the peptide chain of the design target, and In our SEF model, structure properties considered for a single position include secondary structure type, solvent accessibility and backbone Ramachandran torsional angles. Structural properties for a pair of peptide positions include first the above properties associated with individual positions, and second the relative positioning in three-dimensional space of eight atoms at the two positions, including the main chain C, N, α C atoms and the side chain β C atoms. Selecting structure neighbours with adaptive criteria The conditional probability distributions in equations (2) and (3) are to be estimated from the native sequences and structures of training proteins. To extract relevant information from the training proteins, we propose the SSNAC approach that can treat general structural properties such as the relative positioning of a group of atoms in three-dimensional space. To construct the single-residue (or pairwise) SEF terms, every position (or pair of contacting positions) of the target peptide chain is mapped to a target data point in an abstract space spanned by the selected structure properties. Training proteins are treated in the same way: each of their peptide chain positions (or pairs of contacting positions) mapped to a training data point in the same abstract space. Then, the training data points that are neighbours of a target data point can be collected, from which the probability distribution of rotamer types (or pairs of rotamer types) conditioned on the structural properties of the target can be estimated. Based on computational experiments of redesigning single sites in native proteins, the criteria for selecting training residues for a single-residue SEF term have been chosen to be that a selected training residue must have the same secondary structure type as the target residue as well as have backbone torsional angles and solvent accessibilities within certain cutoff distances from those of the target residue. For the pairwise SEF terms, the criteria for selecting training residue pairs comprise; first, the single-residue criteria applied to each of the residues constituting the pair and, second, the selected training residue pair superimposed with the target residue pair using backbone (including β C) atomic coordinates must have a RMSD of atomic positions from the target below a certain cutoff value. The cutoff values in the above scheme are expected to have significant effects on the accuracy of the estimated conditional probability. This accuracy depends on two factors: first, how close the collected training data points are to the target point and, second, how many statistically independent training data points have been collected. The former determines the relevance of the training data and the latter the statistical errors involved. The two factors both depend on the cutoff values, albeit in opposite directions. A key idea of SSNAC is to choose the cutoff criteria adaptively to balance the effects of these two factors on each SEF term. As described in Supplementary Information , for each SEF term, the actual criteria are gradually relaxed in to collect more training data whether a minimum requirement on statistical significance is not met. Correction for small sample effects In conjunction with the SSNAC strategy to select training data, we also developed a procedure to correct the distributions calculated from training data for the effects of small samples. This is especially important for the estimation of the rotamer pair distributions, because there the sample size, that is, the number of training pairs satisfying the criteria for structural neighbours, can be especially small relative to the number of possible pair types. Here we use the rotamer pair distribution for a position pair ( i, j ) as an example to illustrate the correction. Let N be the sample size and k(r i , r j ) the number of training pairs of rotamer pair type (r i , r j ). If the ‘true’ probability of the pair (r i , r j ) is p , the likelihood of p given the observed values of N and k (i.e. the probability of observing ( r i , r j ) for k times in N samples) can be calculated as .This likelihood is maximized with respect to p when p = p obs ( r i , r j )= k ( r i , r j )/ N , yielding Based on L max , we can define ‘an interval of high confidence’, [ p low , p high ], for p around p obs ( r i , r j ), with the bounds p low and p high determined by Next, we estimate p as a weighted sum of p obs ( r i , r j ) and a ‘background’ probability p bg , namely, The background probability is obtained by neglecting any pairwise interaction, that is, The weighting factor α is determined by The rational behind equation (7) is that it weights the background probability more when the observed probability involves a larger uncertainty, while shifting towards the observed probability when the confidence interval becomes narrower relative to the background probability. Beyond this rational, formula (7) has been chosen empirically, trial calculations using single site redesign involved. The final estimation of the probability is Normalization of the estimated probabilities can be done after all possible rotamer pair types have been considered, not affecting the relative SEF energies. Van der Waals interactions The purely statistical pairwise terms represent the inter-residue packing with coarse-grained rotamers. An extension to explicitly include atomic van der Waals interactions with finer rotamers has been considered. This leads to a modified total energy of the form (see also Supplementary Method and Supplementary Table 4 ). At the current stage, it is still unclear whether the extended E SEF_v can indeed improve over the purely statistical E SEF in protein design, so both energy functions have been used to design sequences that were subjected to theoretical and experimental tests. For the experimentally studied proteins, those designed with E SEF have been named as ‘D_X’ and those designed with E SEF_v named as ‘Dv_X’, the symbol ‘X’ to be replaced by the PDB ID of the actual target. The amino acid sequences of these proteins are given in Supplementary Table 10 . Single-site redesign Following Kuhlman et al. [4] , we mainly employed single-site redesign experiments to guide the parameterization of the energy functions. More details about the derivation and implementation of the energy functions can be found in Supplementary Information . Energy minimization A simple Metropolis Monte Carlo-simulated annealing approach has been used to minimize the sequence energy functions. Each simulation started from a random initial sequence and a high temperature that was gradually lowered subsequently. The simulation ended when no rotamer change has been accepted for a long period. The rate of annealing depended on sequence length, and has been chosen so that different initial sequences could converge to similar final sequences that were not only of high mutual sequence identity (above 80%) but also of variance in their energies only a few tenths of the energy differences between the designed sequences and the native sequences. For energy evaluations of given amino acid sequences, the same simulated annealing process was applied to obtain a E SEF or E SEF_v minimized with respect to varying the rotamer types with fixing amino acid types. There the global minimum could be found with different simulation runs converged to exactly the same results. Calculations using Rosetta The Rosetta 3.2 programme package has been obtained from https://www.rosettacommons.org/ . Fixed backbone designs have been carried out by running ‘fixbb.linuxgccrelease’ with recommended default parameters. Ab initio structure predictions have been performed by running ‘AbinitioRelax.linuxgccrelease’ with the following example flags set in input: -database rosetta-3.2/rosetta_database -in:file:fasta 1q1fA.fasta -in:file:frag3 aa1q1fA03_05.200_v1_3 -in:file:frag9 aa1q1fA09_05.200_v1_3 -abinitio:relax -relax:fast -abinitio::increase_cycles 10 -abinitio::rg_reweight 0.5 -abinitio::rsd_wt_helix 0.5 -abinitio::rsd_wt_loop 0.5 -use_filters true -psipred_ss2 1q1fA.psipred_ss2 -out:nstruct 200 -out:pdb To evaluate the Rosetta energies of a given sequence for a given target structure, we first ran ‘fixbb.linuxgccrelease’ with the amino acid types at all positions fixed to obtain an initial structure with frozen backbone and optimized side-chain conformations. Then the entire structure was relaxed by running ‘relax.linuxgccrelease’ with the value of flag ‘ relax ’ set as ‘ fast ’. Protein preparation and structure characterization First, DNA sequences encoding the proteins were synthesized and cloned into a modified pET-28a(+) vector by using the NdeI and XhoI sites. Proteins expressed and purified from cells of the Escherichia coli strain Rosetta were used for NMR and CD studies. NMR experiments were performed at 298 K on a Bruker DMX500 or DMX600 spectrometer equipped with triple resonances, self-shielded z axis gradient probes. Data were processed using the programmes NMRDraw/NMRPipe [32] . Spectra were analysed and assigned using the programme SPARKY 3 (ref. 33 ). The Program Procheck [34] was used to assess the overall quality of the structure. In terms of structure calculations for Dv_1ubq and D_1cy5_M2, the details of the input restraints and structural statistics are presented in Supplementary Table 11 . For each protein, 20 refined structures are shown in Supplementary Fig. 6 . Thermally induced denaturation of designed proteins under different conditions were evaluated by DSC using a VP-DSC Microcalorimeter (Microcal) in a 0.509-ml cell at a heating rate of 1 °C min −1 . Before the measurements, the sample and the reference were degassed at 10 °C for 15 min. The Dv_1ubq protein concentration was 10 mg ml −1 in PBS buffer, D_1cy5_M1 and D_1cy5_M2 concentrations were 4 mg ml −1 in PBS buffer and Dv_1r26_M1 concentration was 1 mg ml −1 in 10 mM KH 2 PO 4 , 100 mM KCl buffer. The thermograms were background-corrected and normalized to the molar concentration. The lower concentration for Dv_1r26_M1 had to be used to avoid the problem of protein aggregation on thermalization, although it led to lower signal-to-noise ratios in results (see Supplementary Fig. 1 ). CD data were collected on a Jasco-810 spectrophotometer. Chemical-induced denaturation of native ubiquitin and of designed Dv_1ubq with GuHCl was monitored at 222 nm for 0.2–0.4 mg ml −1 protein samples in 10 mM NaH 2 PO 4 , 100 mM NaCl buffer at 25 °C in a 1 mm path-length quartz cuvette. Far-ultraviolet CD spectra of Dv_1ubq, D_1cy5_M1, D_1cy5_M2 and Dv_1r26_M1 were measured from 200 to 260 nm for 0.2 mg ml −1 protein samples in 10 mM KH 2 PO 4 , 100 mM KCl buffer at various temperatures of 25, 50, 75 and 95 °C in a 1-mm path-length cuvette. The thermal denaturation CD data were obtained by measuring ellipticity every 5 °C of temperature increasing from 25 °C to 95 °C at λ =218 nm (for Dv_1ubq and Dv_1r26_M1) or λ =222 nm (for D_1cy5_M1 and D_1cy5_M2). Antibiotics resistance measurements Sequence of interest flanked by linker sequences of repetitive glycines and serines were introduced into TEM1-β-lactmase using the vector pMB1-tet-pARA-bla-link_long (LFM10, courtesy of Dr Bardwell). Mid-log phase cells expressing TEM1-β-lactamase containing inserted guest proteins were normalized to A 600 =1. Two microlitres of serial dilutions of cultures from 10 0 to 10 −6 were spotted on LB plates containing 2.0 mg ml −1 of ampicillin. After 18 h incubation at 37 °C, growth or no growth for different dilutions was examined. Directed evolutions Random mutagenesis was achieved through error-prone PCR [35] , the products of which were used to construct plasmid libraries using MEGAWHOP cloning [36] or ligation with the LFM10 vector digested with BamHI/XhoI. Each directed evolution round selected from a capacity of 10 5 –10 6 colonies and the load of error-prone PCR random mutations was kept accordingly low. LB plates containing 1.0, 1.5 or 2.0 mg ml −1 of ampicillin were used for selection. The colonies showing the highest antibiotics resistance were selected and verified by re-cloning the target sequence segments into the original LFM10 vector followed by antibiotics resistance assay with serial dilution [23] . Accession codes: Atomic coordinates of the structures of Dv_1ubq and D_1cy5_M2 have been deposited in the PDB under accession code 2MLB and 2MN4 , respectively. How to cite this article: Xiong, P. et al. Protein design with a comprehensive statistical energy function and boosted by experimental selection for foldability. Nat. Commun. 5:5330 doi: 10.1038/ncomms6330 (2014).